The future of low-temperature carbon dioxide electrolysis depends on solving one basic problem 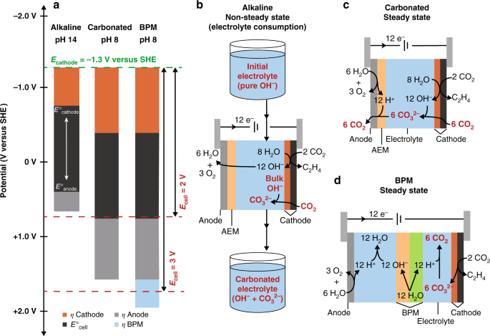Fig. 1: The CO32–problem. aVisualization of various contributors to the cell voltage for a CO2electrolysis cell operating under alkaline conditions, carbonated conditions, or with a bipolar membrane (BPM). The contributions shown are the thermodynamic cell potential (E°cell), and cathode, anode, and BPM overpotentials (η). Electrode potentials are referenced to the SHE scale. For simplicity, cell resistance was not included, which would add to the cell voltage. The green dotted line represents the least negative cathode potential reported for low-temperature CO2reduction at >200 mA cm–27. The red dotted lines provide a visual reference for cell voltages. The thermodynamic potentials for the cathode (E°cathode) and anode (E°anode) shift positive versus SHE as the pH is decreased. Alkaline conditions minimize cell voltage but cannot be maintained at steady state because of CO32–formation.bSchematic of anion transport in an alkaline flow cell showing OH–consumption by CO2.cSchematic of a cell at steady state after carbonation showing the carbon loss due to CO2released at the anode.dSchematic of a BPM cell at steady state. Hydroxide consumption makes alkaline CO 2 electrolyzers fuel-wasting devices The state-of-the-art for low-temperature CO 2 electrolysis has been obscured by studies that utilize a reservoir of flowing alkaline electrolyte to maintain a high pH in the cell [5] , [6] , [7] , [8] . High pH minimizes the cell voltage, which makes these systems appear to have high energy efficiency, but consumption of OH – in the reservoir by CO 3 2– formation results in a net negative energy balance. Understanding why the cell voltage is minimized at high pH helps to clarify the CO 3 2– problem (Fig. 1a ). For most known catalyst materials, including Au and Cu, the CO 2 reduction rate depends on the electron transfer driving force but not explicitly on pH [9] , [10] , [11] , [12] , [13] . As a result, synthetically relevant current densities require rather negative potentials versus an absolute reference such as the standard hydrogen electrode (SHE). Even with high surface area electrodes, CO 2 reduction at a geometric current density of >200 mA cm –2 has generally required potentials <–1.3 V versus SHE. Because the thermodynamic electrode potentials become more negative versus SHE as the pH is increased, the cathode overpotential is minimized by increasing pH at a fixed cathode potential versus SHE. The overpotential for oxygen evolution at the anode is also generally lowest in base. These contributions significantly reduce the cell voltage at high pH (Fig. 1a ). Fig. 1: The CO 3 2– problem. a Visualization of various contributors to the cell voltage for a CO 2 electrolysis cell operating under alkaline conditions, carbonated conditions, or with a bipolar membrane (BPM). The contributions shown are the thermodynamic cell potential ( E ° cell ), and cathode, anode, and BPM overpotentials ( η ). Electrode potentials are referenced to the SHE scale. For simplicity, cell resistance was not included, which would add to the cell voltage. The green dotted line represents the least negative cathode potential reported for low-temperature CO 2 reduction at >200 mA cm –2 [7] . The red dotted lines provide a visual reference for cell voltages. The thermodynamic potentials for the cathode ( E ° cathode ) and anode ( E ° anode ) shift positive versus SHE as the pH is decreased. Alkaline conditions minimize cell voltage but cannot be maintained at steady state because of CO 3 2– formation. b Schematic of anion transport in an alkaline flow cell showing OH – consumption by CO 2 . c Schematic of a cell at steady state after carbonation showing the carbon loss due to CO 2 released at the anode. d Schematic of a BPM cell at steady state. Full size image While minimizing cell voltage is obviously desirable, cells operating under flowing alkaline conditions are not at steady state. The OH – in the electrolyte reservoir is continuously consumed by exergonic CO 3 2– formation as it contacts CO 2 at the cathode (Eq. 1 [14] and Fig. 1b ): 
    2OH^-_(aq) + CO_2(g)→CO_3^2 - _(aq) + H_2O_(l) ΔG^∘ = -56 kJ mol^-1
 (1) In practice, the energy required to regenerate CO 2 and 2 OH – from aqueous CO 3 2– is much larger than |Δ G °|, for example >230 kJ mol –1 with an optimized system using a calcination cycle [15] . Depending on the product, the energy stored by CO 2 electrolysis is ~100–130 kJ mol –1 of electrons. Thus, the energy balance with flowing alkaline electrolyte will be negative if carbonation consumes ~1 OH – equivalent for each electron of CO 2 electrolysis current. Though it is rarely quantified, one recent study reported that ~3 OH – were consumed per electron of CO 2 -to-CO electrolysis current with a flowing 1 M KOH electrolyte [8] . Unfortunately, it is common practice to ignore OH – consumption and calculate an “energy efficiency” based solely on the applied voltage, thermodynamic voltage, and faradaic efficiency. These values are qualitatively incorrect. In reality, flowing alkaline CO 2 electrolysis cells are fuel-wasting devices because it would require more fuel to regenerate the spent electrolyte than the amount of fuel produced by the electrolysis. Using data from flowing alkaline conditions in technoeconomic analyses will grossly overestimate the state-of-the-art for CO 2 electrolysis. Conversion of power to fuel with a positive energy balance requires operating under steady state conditions where there is no net electrolyte consumption. In a cell operating at steady state, CO 3 2– is still formed continuously at the cathode by reaction of CO 2 with the electrogenerated OH – , but it is protonated elsewhere in the cell to release CO 2 . In an anion-transporting cell such as an anion exchange membrane (AEM) cell, CO 3 2– is transported to the anode (Fig. 1c ). In order to protonate CO 3 2– , the anode pH equilibrates to near-neutral (pH ~ 8) [2] , which increases the cell voltage compared to high pH because the anode thermodynamic potential moves in the positive direction (Fig. 1a ). In addition, there is a much greater oxygen evolution overpotential at near-neutral pH with available catalysts. Thus, most of the energy penalty from the CO 3 2– problem is a consequence of what happens at the anode. In fact, the same problem is seen in AEM water electrolysis, where the cathode catalyzes H 2 evolution. Contamination of an AEM water electrolyzer with trace amounts of air (400 ppm CO 2 ) results in the formation of CO 3 2– , which causes a >1 V increase to the cell voltage [16] . The steady state carbon flux imposed by CO 3 2– formation also sets an upper limit on carbon efficiency in anion transporting cells. For CO 2 reduction to CO, one CO 2 is released at the anode for every CO that is produced at the cathode, resulting in a maximum carbon efficiency of 50%. For ethylene, the maximum is 25% (Fig. 1c ). Many cells operate at much lower carbon efficiencies than these maxima because a large excess of CO 2 is supplied to the cathode to support high current densities. Low carbon efficiency is a major barrier to large-scale chemical and fuel electrosynthesis because there is a substantial energy and financial cost to obtain a CO 2 feedstock of suitable purity. An alternative to an anion transporting cell is to operate with a bipolar membrane (BPM) configured such that CO 2 electrolysis is coupled with water dissociation at the BPM. At steady state, CO 3 2– generated at the cathode is protonated at the BPM interface, releasing CO 2 on the cathode side (Fig. 1d ). While this design avoids releasing CO 2 at the anode [17] , it has a lower energy efficiency than an AEM cell because the BPM imposes an additional overpotential in order to drive water dissociation (Fig. 1a ). It is important to note that CO 2 crossover through a BPM is low but non-zero [18] . As such, BPM cells that start with high pH on the anode side will transform to a CO 3 2– electrolyte at steady state. The consequences of the CO 3 2– problem are evident in the performance that has been demonstrated at steady state. For the production of CO, the best reported performance is for lab-scale (5 cm 2 ) devices that have been operated at steady state for >4000 h at ~200 mA cm –2 CO 2 -to-CO current density, nicely demonstrating the viability of durable CO electrosynthesis at a reasonable rate. However, the carbon efficiency is 50% and the cell voltage is 3.0 V, corresponding to an energy efficiency of only 43% [1] , [19] . Both of these values are consistent with the analysis in Fig. 1 . To make a more reduced product such as ethylene, the CO 3 2– problem is more pronounced. The best reported performance at steady state is 60 h of operation at ~500 mA cm –2 CO 2 -to-ethylene current density, ~2% carbon efficiency, and a cell voltage of 3.9 V, corresponding to an energy efficiency of ~15% [20] . The evaluation of full cell metrics under steady state conditions remains uncommon in CO 2 electrolysis research, but such experiments are essential for assessing progress and should become standard to demonstrate the impact of a material or design advance. Low-temperature CO 2 electrolysis will not be competitive with other electrical energy storage or CO 2 conversion technologies without major gains in energy and carbon efficiency. Reducing the overpotential of CO 2 reduction catalysis remains an important objective provided it can be realized under steady state conditions at high current density. Avoiding the losses imposed by CO 3 2– formation demands a much broader research effort that includes strategies to control the formation and clearance of CO 3 2– , creative cell designs, and far greater attention to the anode. The progress on the CO 3 2– problem will determine the trajectory of CO 2 electrolysis in the next 10 years and its impact beyond the laboratory.